Symmetry-protected topological phases from decorated domain walls Symmetry-protected topological phases generalize the notion of topological insulators to strongly interacting systems of bosons or fermions. A sophisticated group cohomology approach has been used to classify bosonic symmetry-protected topological phases, which however does not transparently predict their properties. Here we provide a physical picture that leads to an intuitive understanding of a large class of symmetry-protected topological phases in d =1,2,3 dimensions. Such a picture allows us to construct explicit models for the symmetry-protected topological phases, write down ground state wave function and discover topological properties of symmetry defects both in the bulk and on the edge of the system. We consider symmetries that include a Z 2 subgroup, which allows us to define domain walls. While the usual disordered phase is obtained by proliferating domain walls, we show that symmetry-protected topological phases are realized when these domain walls are decorated, that is, are themselves symmetry-protected topological phases in one lower dimension. This construction works both for unitary Z 2 and anti-unitary time reversal symmetry. Symmetry-protected topological (SPT) phases are gapped quantum phases with topological properties protected by symmetry [1] . The ground states of SPT phases contain only short-range entanglement and can be smoothly deformed into a totally trivial product state if the symmetry requirement is not enforced in the system. However, with symmetry, the nontrivial SPT order is manifested in the existence of gapless edge states on the boundary of the system that cannot be removed as long as symmetry is not broken. Many SPT phases have been discovered over the past decades [2] , [3] , [4] , [5] , [6] , [7] , [8] , [9] , [10] , [11] , [12] , [13] , [14] , [15] , [16] , [17] , [18] , [19] , [20] , [21] , [22] and a general structure of the theory of SPT phases is emerging. In 1d, SPT phases have been completely classified for general interacting bosonic/fermionic systems that carry nontrivial projective representations of the symmetry in their degenerate edge states [23] , [24] , [25] . In fact, the Haldane/AKLT phase of spin-one quantum antiferromagnet is a physical realization of a one-dimensional (1D) SPT phase, which is protected by spin rotation or time reversal symmetries. Two-dimensional (2D) SPT phases were first discovered in topological insulators and superconductors, which have subsequently been generalized to three dimensions [26] , [27] , [28] . Such free fermion SPT phases have been realized experimentally [29] , [30] , [31] , [32] and also classified completely for systems with internal symmetries [33] , [34] , [35] . Classification of free fermion SPT phases with spatial symmetries is not complete yet but a lot of progress has been made, see for example, refs 36 and 37 . Recently, it was realized that two- and higher-dimensional SPT phases exist not only in free fermion systems but also in strongly interacting boson systems, and a systematic construction is given based on the group cohomology of the symmetry [1] . While the construction provides a fixed point description in the bulk, it is hard to access edge dynamics and hence how the system responds to physical perturbations. Also it is not clear in what physically realistic systems can these bosonic SPT phases be realized. Much progress has been achieved recently in understanding the low energy physics and finding physical realizations for some of the bosonic SPT phases. In 2D, a general understanding of SPT phases with Abelian (and time reversal) symmetry has been given in terms of Chern–Simons K-matrix theory [6] , which also provides a field theory of the protected edge states. A physical realization of the U (1) SPT phases (which are expected to have even integer-quantized quantum Hall conductance [6] ) has been proposed in bosonic cold atom systems with artificial gauge fields [8] . The 2D SPT phases with nonabelian SO (3) and SU (2) symmetry was studied with nonlinear sigma model with quantized topological θ terms and are found to have quantized spin transport [13] . More recently, some three-dimensional (3D) SPT phases have been understood within a field theoretic approach, which predicts surface vortices with projective representations and quantized magnetoelectric responses [9] . Recently, 3D SPT phases have been discussed from number of different theoretical perspectives, including twisted vortex condensates [18] and the statistical magneto-electric effect [20] . A useful perspective on SPT phases appears on gauging the symmetry discussed by Levin and Gu [5] in 2D, and recently extended in other studies [20] , [21] , [38] , [39] , [40] to 3D phases. Finally, we note a special feature of 3D SPT phases is that their surface states could be gapped and fully symmetric if they develop topological order just at the surface [9] , [20] , [21] , [22] . In this paper, we focus on SPT phases with symmetry group Z 2 × G and present a simple construction of d dimensions SPT phases by decorating the domain walls of Z 2 configurations in the bulk with d −1 dimensional SPT states with G symmetry. Such a construction naturally reveals some of the special topological features of such phases. For example, it is easy to see that when a domain wall is cut open at the boundary of the system, the end points/loops of the domain wall carry gapless edge states of the d −1 dimensional SPT state with G symmetry. The same is true on the flux point/loops in the system when the Z 2 part of the symmetry is gauged. In particular, in the Result section we are going to present the construction of a 2D SPT phase with symmetry by decorating the 1D Z 2 domain walls with Haldane chains and a 3D SPT phase with Z 2 × Z 2 symmetry by decorating the 2D Z 2 domain walls with the nontrivial 2D SPT phase with Z 2 symmetry. Supporting numerical evidence and generalizations of our results are presented in the Methods section, which include numerical analysis of symmetry on the edge of the 2D SPT phase with symmetry, discussion of gauging the Z 2 symmetry and the construction of a 1D SPT phase with Z 2 × Z 2 symmetry and 3D SPT phases with , and symmetries. These results are summarized in Figs 1 , 2 , 3 . The relation between the domain wall construction and the Künneth formula for group cohomology is also discussed in the methods section. Brief reviews of the group cohomoloy description of SPT phases, the field theory description of 2D and 3D SPT phases are given in the Supplementary Material . 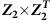Figure 1: SPT phase in 2D withZ2and time-reversal symmetry (). A snapshot of the ground state wave function: blue and grey are oppositely directed domains of theZ2symmetry. The ground state preserves theZ2symmetry since it is a superposition of domain configurations. The domain walls themselves (black lines) are in ad=1 SPT phase (the Haldane/AKLT phase) protected by time reversal symmetry. When they end at the edge of the system they create Kramers doublets, leading to a gapless edge state. Figure 1: SPT phase in 2D with Z 2 and time-reversal symmetry ( ). A snapshot of the ground state wave function: blue and grey are oppositely directed domains of the Z 2 symmetry. The ground state preserves the Z 2 symmetry since it is a superposition of domain configurations. The domain walls themselves (black lines) are in a d =1 SPT phase (the Haldane/AKLT phase) protected by time reversal symmetry. When they end at the edge of the system they create Kramers doublets, leading to a gapless edge state. 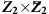Figure 2: SPT phase in 3D withsymmetry. Red (blue) surfaces represent domain walls of theZ2() symmetry. They intersect along curves (black lines). The ground state wave function is a superposition of all domain wall configurations that differ by a sign depending on whether there is an even or odd number of intersection curves. This automatically implies a protected edge state when a domain wall intersects the surface of the sample (grey dashed line). Full size image Figure 2: SPT phase in 3D with symmetry. Red (blue) surfaces represent domain walls of the Z 2 ( ) symmetry. They intersect along curves (black lines). The ground state wave function is a superposition of all domain wall configurations that differ by a sign depending on whether there is an even or odd number of intersection curves. This automatically implies a protected edge state when a domain wall intersects the surface of the sample (grey dashed line). 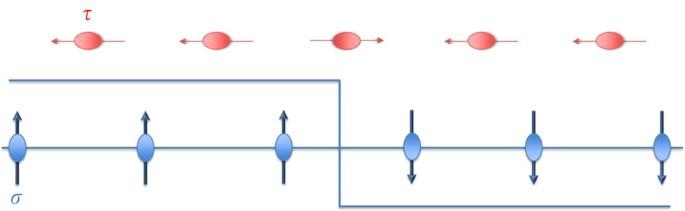Figure 3: An SPT phase in 1D protected byZ2×Z2symmetry. This phase involves two sets of spinsσ,τand emerges from the ordered phase of theσspins by condensing domain walls attached to spin flip excitations of theτspins. Full size image Figure 3: An SPT phase in 1D protected by Z 2 × Z 2 symmetry. This phase involves two sets of spins σ , τ and emerges from the ordered phase of the σ spins by condensing domain walls attached to spin flip excitations of the τ spins. Full size image 2D SPT phase with symmetry Let’s start with the simplest example in this construction: a 2D SPT phase with symmetry where represents time reversal symmetry. Intuitively, the state is constructed by attaching 1D Haldane chains with time-reversal symmetry to the domain walls between Z 2 configurations on the plane and then allow all kinds of fluctuations in the domain wall configurations. With such a structure, it is then easy to see that when the system has a boundary where domain walls can end, the end point would carry a spin 1/2 degree of freedom (edge state of Haldane chain) that transforms projectively under time reversal. First, we describe a 2D lattice wave function of the ground state that is gapped and does not break any symmetry. Then, we discuss what happens on the boundary of the system. By identifying the relation between symmetry action on the edge and the nontrivial cocycle of symmetry group, we establish the existence of nontrivial SPT order in this model. It is known that this SPT phase with symmetry can be described with U (1) × U (1) Chern–Simons theory with a nontrivial symmetry action. We review this description and demonstrate the nontrivial topological feature of domain walls in the field theory language. Bulk wave function on 2D lattice Consider a honeycomb lattice as shown in Fig. 4a where each plaquette hosts a Z 2 variable (big black dot) in state |0 or |1 . The Z 2 part of the symmetry flips |0 into |1 and |1 into |0 . At each vertex, there are four spin 1/2’s (one at the center and three on links as shown in Fig. 4b ). On each spin 1/2 time-reversal symmetry acts as = iσ y K and satisfies 2 =−1. On the total Hilbert space of each vertex, time reversal still satisfies 2 =1 and forms a linear representation of . Now consider a Hamiltonian term that enforces that in the ground state two spin 1/2’s on the same link form a time-reversal singlet pair if the link is on a Z 2 domain wall while the remaining spin 1/2’s that are not on a domain wall form singlets within each vertex (there is always an even number of these at each vertex). For the vertex that is not on a domain wall, we can put the four spins into the symmetric total singlet state. The effect of this term can be thought of as attaching Haldane chains to all the Z 2 domain walls. A possible configuration in the ground state is shown in Fig. 4c where the dotted lines represent singlet pairing. Note that while the Haldane chain is usually defined in spin-1 systems, here for simplicity of discussion we use the fixed point form of the wave function where each spin-1 is replaced with two spin-1/2’s. A tunneling term between the configurations is then added to the Hamiltonian that in the low energy sector of flips the Z 2 variables together with the related singlet configurations. flips the Z 2 spin in a plaquette and i flips the Haldane chain configuration around it. P projects onto the low energy sector of . Figure 5 illustrates one term in . 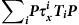Figure 5: One term in. Two spin ½’s connected by dotted lines are in the singlet state, four spin ½’s connected by dotted lines are in the symmetric total singlet state, arrows denote the state of unpaired spin ½’s, which are preserved in the flipping. 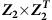Note that when flipping a segment of the Haldane chain from one side of the plaquette to another side, the state of the edge spin 1/2’s are preserved. Figure 4: Two-dimensional SPT model withsymmetry. Lattice model: (a) each plaquette hosts aZ2variable (big black dot) (b) each vertex hosts four spin ½’s (small blue dots) (c) two spin ½’s on the same link form a singlet if they are on aZ2domain wall, other spin ½’s form singlets within each vertex. Figure 4: Two-dimensional SPT model with symmetry. Lattice model: ( a ) each plaquette hosts a Z 2 variable (big black dot) ( b ) each vertex hosts four spin ½’s (small blue dots) ( c ) two spin ½’s on the same link form a singlet if they are on a Z 2 domain wall, other spin ½’s form singlets within each vertex. Full size image Figure 5: One term in . Two spin ½’s connected by dotted lines are in the singlet state , four spin ½’s connected by dotted lines are in the symmetric total singlet state , arrows denote the state of unpaired spin ½’s, which are preserved in the flipping. Full size image The V k terms and the terms are local and commute with each other. The ground state of the total Hamiltonian is exactly solvable and is an equal-weight superposition of all possible consistent configurations of Z 2 variables and singlets. The ground state is unique, gapped and preserves symmetry. To see this, note that to each domain wall configuration there is a unique state of the spins that live at the vertices. This is enforced by the first term in the Hamiltonian in equation (1) that projects into the manifold of states that follow this association. In the absence of any decoration, the equal superposition of domains is the ground state of . Now, in order that the decorated spin configurations are properly generated, one induces the same matrix elements between domain wall configurations as , but where each domain wall configuration appears along with its unique spin state attached. Let us denote these operators as . Since these only affect the spins near the flipped bit, they are local operators and take the form of the second term in the Hamiltonian in equation (1). Moreover, they are readily seen to commute with one another and the constraint, when acting within the low energy manifold, since they essentially mimic the action of the , with the decorating spin configuration simply coming for the ride. Edge state Interesting things happen when the system has a boundary. When the system is cut open, the Z 2 domain walls will have end points on the boundary. As the spin singlets are tied to domain walls in the bulk, on the boundary there will be isolated spin 1/2’s on the end points of Z 2 domain walls. Imagine that we cut the system through the middle of plaquettes (In order not to cut through degrees of freedom, we can first split the Z 2 variable into two, one on each side of the cut and add a Hamiltonian term for them to be equal. This does not violate the symmetry of the system and is therefore allowed). The 1D boundary degrees of freedom then contain two parts: the bond Z 2 variables that come from plaquettes on the cut and the vertex spin variables when the neighboring bonds contain different Z 2 configurations, as shown in Fig. 6a . Symmetry acts by flipping the Z 2 variable and time-reversing the spins. 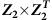Figure 6: Two equivalent descriptions of the boundary of 2D SPT model withsymmetry. (a) thick bonds representZ2variable in stateand thin bonds, spin 1/2 exists on their domain wall. (b) OneZ2variable per bond and one spin variable per vertex. Time reversal acts on spins in a way dependent of neighboringZ2configurations. Dotted boxes represent local degrees of freedom on the 1D boundary labelled by group elements. Figure 6: Two equivalent descriptions of the boundary of 2D SPT model with symmetry. ( a ) thick bonds represent Z 2 variable in state and thin bonds , spin 1/2 exists on their domain wall. ( b ) One Z 2 variable per bond and one spin variable per vertex. Time reversal acts on spins in a way dependent of neighboring Z 2 configurations. Dotted boxes represent local degrees of freedom on the 1D boundary labelled by group elements. Full size image To study the boundary as an effective 1D, we will use a slightly different description of the boundary degrees of freedom. In the previous description, the existence of vertex degrees of freedom are dependent on the bond degrees of freedom. Equivalently, we can also think of the boundary as a local 1D system with independent degrees of freedom on the bonds and the vertices, as shown in Fig. 6b . That is, we can imagine that there exist pseudo-spins (empty circles) on the vertices when neighboring Z 2 variables are the same. On the pseudo-spins time reversal acts simply as = σ x K and satisfies 2 =1. The pseudo-spin can be thought of as the direct sum of two spin-0 dimensions |0 +|1 and i (|0 −|1 ). The total symmetry action is then It is easy to see that such a description of the boundary can be reduced to the previous one by polarizing each pseudo-spin in the z direction. As 2 =1 on each pseudo-spin, polarizing them does not break time-reversal symmetry. Using this description, we can see explicitly how this model is related to the nontrivial third cocycle of the symmetry group and therefore contains nontrivial SPT order. We can also write down effective Hamiltonians for the boundary and solve for the low-energy dynamics, as we demonstrate in the following. In terms of the local degrees of freedom on the 1D edge state, σ and τ , the Z 2 symmetry action on the edge reads and time reversal acts as We can write down an effective Hamiltonian satisfying the symmetry and solve for the dynamics on the 1D edge. Some simple interaction terms that satisfy both the Z 2 symmetry (equation 2) and the time-reversal symmetry (equation 3) include and . Therefore, a possible form of the dynamics of the edge is given by Hamiltonian This Hamiltonian can be mapped exactly to an XY model by applying unitary transformations to each pair of τ i and σ i variables. The Hamiltonian that we get after these transformations is and the symmetry transformations are mapped to and In order to see how the symmetry acts on the low-energy effective theory, we diagonalize the XY Hamiltonian , identify the free boson modes in the low energy eigenstates and calculate the action of the symmetry on the low-energy states. The low-energy states are labelled by quantum numbers n k ∈ Z and , k =0, 1, 2…, where n 0 and label the total angular momentum and the winding number of the boson field respectively and n k and , k >0, label the left/right moving boson modes. The Z 2 symmetry acts by mapping state to and time-reversal symmetry acts by mapping state to , which is consistent with the low-energy description given in the next section where Z 2 symmetry acts as ϕ 1 →− ϕ 1 , ϕ 2 →− ϕ 2 and time-reversal acts as ϕ 1 →− ϕ 1 +π, ϕ 2 → ϕ 2 +π on the chiral boson fields { ϕ 1,2 }. Effective field theory description As discussed in ref. 6 , SPT phases in 2D may be characterized by the unusual transformation properties of their edge states, under the action of symmetry. The simplest situation, which captures a large fraction of SPT phases, is a Luttinger liquid edge with a single gapless bosonic mode. The edge fields are characterized by compact conjugate bosonic fields ϕ 1 , ϕ 2 such that Physically, inserts a boson at point x along the edge, while inserts a phase slip. We see that the 2D SPT phase of interest implies the following transformation law: This is different from the form we discussed in the last section. However, as we show in the Supplementary Note 3 and 4 , these two forms are actually equivalent to each other. Note, this edge cannot be gapped out without breaking symmetry. Terms that gap the edge such as cos ϕ 1,2 are forbidden by symmetry. If either one of the symmetries is broken, then a trivial edge is possible. Finally, let us verify that a domain wall of the Z 2 order, terminating at the edge carries a Kramer’s pair, as the pictorial description implies. The operator that creates a domain wall, rotates ϕ 1 by π everywhere (say) to the right of the point x . By the commutation relation 8, this is identified with the operator Now, let us consider how the domain wall insertion operator transforms under time reversal . In particular, we would like to calculate the action of acting twice with time reversal and see whether 2 =±1. Now . Applying this again we find: thus, we find that for this operator 2 =−1. Hence, it must carry a Kramer’s degeneracy as expected from the physical picture. Connection to group cohomology Now let us establish the nontrivial SPT order in this state by identifying the connection of the symmetry actions on the boundary with nontrivial third cocycles. When we think of the boundary as a local 1D system with independent bond variables and vertex variables (that is, treating spins and pseudo-spins as equivalent variables), symmetry no longer acts on the degrees of freedom independently. The Z 2 part of the symmetry still acts on each Z 2 variable independently. However, time-reversal symmetry on the vertices depends on the Z 2 configurations on the bonds, as shown in equation (3). This is exactly the signature of SPT phases. Indeed, as was shown in ref. 1 , the boundary of d D STP phases can be thought of as a d −1D local system where the symmetry acts in a non-onsite way. Without symmetry, the boundary can be easily gapped out. If the symmetry acts in an on-site way, the boundary can be simply gapped out by satisfying the symmetry on each site. However, with non-onsite symmetry related to nontrivial group cocycles, the boundary must remain gapless as long as symmetry is not broken. In particular, in the group cohomology construction as reviewed in the Supplementary Note 2 , the boundary local degrees of freedom are labelled by group elements α i of the symmetry group and the action of the symmetry operator involves two parts: first, changing the local states | α i to | αα i ; second, multiplying a phase factor given by nontrivial cocycles to each pair of α i and α i +1 . More specifically, on the 1D boundary of 2D SPT phases, the symmetry acts as where f α ( α i , α i +1 ) is a phase factor given by the nontrivial third cocycle ω 3 Now we can show that the symmetry action on the boundary of the model we constructed is of exactly this form. We can consider the pair of Z 2 variables α i =( τ i , σ i ) (dotted box in Fig. 6b ) as labelling group elements in the group . That is, we consider the Z 2 state |0 /|1 of τ as labelling the trivial/nontrivial element in group Z 2 and the spin state |↑ /|↓ of σ as labelling the trivial/nontrivial element in group . Then, the Z 2 part of the symmetry is the following mapping and the time-reversal part of the symmetry (given by either = σ x K on the pseudo-spin or = iσ y K on the spin) also involves the mapping Therefore, a general symmetry operation labelled by α =( τ , σ ), τ ∈ Z 2 , , will first change group elements labels in each box Moreover, the time-reversal symmetry also adds a (−1) phase factor when the neighboring Z 2 variables are different and when the vertex variable was originally in state |↑ . Such a phase factor on spin σ i can be written as Here σ z =1 in |↑ , σ z =−1 in |↓ and τ z =1 in |↑ , τ z =−1 in |↓ . Therefore, the symmetry action on the boundary can be put exactly into the form of equation (12) with when the symmetry action α involves time reversal and when α does not involve time reversal. We can reorganize the variables and write the phase factor as a function of , It can be checked that is a nontrivial third cocycle of group , using the cocycle conditions introduced in the Supplementary Note 1 . Therefore, we can show using methods in ref. 3 that the boundary must be either gapless or symmetry breaking and the 2D bulk is in a nontrivial SPT phase. 3D SPT phase with Z 2 × Z 2 symmetry Now we go one dimension higher and consider the Z 2 × Z 2 group. To differentiate the two Z 2 ’s, we write them as Z 2 and . We can start with similar constructions in the bulk where the nontrivial SPT phase in two dimension is attached to the domain wall of the Z 2 configuration in the cubes. A simple understanding of the ground state wave function exists starting from Levin and Gu’s [5] construction of 2D SPT phase with Z 2 symmetry. It was shown that in the 2D SPT model the ground state wave function takes the simple form of where N C is the number of domain walls in configuration . Such a wave function has gapless edge states when the system has a boundary. Now consider the symmetry . This has elements {1, g 1 , g 2 , g 3 }. We will pick two of the three nontrivial elements say g 1 , g 2 . Choose any one of these two generators (say g 1 ) and consider domain walls in 3D between regions that break this symmetry in opposite ways. This defines closed 2D manifolds. Now, on these closed manifolds the domain walls of the second generator ( g 2 ) are examined and number of closed loops counted (essentially these loops are intersections of domain walls of g 1 and g 2 ). Now, one uses this set of closed loops and defines a wave function as in equation (21). This is the wave function of a symmetric state where is the number of closed loops formed by the intersection of the g 1 and g 2 domain walls in configuration (see Fig. 2 ). What is the physical consequence of this wave function? Consider breaking one of the Z 2 symmetries and forming a domain wall (of say g 1 ). Now, the domain wall is the edge state of the 2D SPT phase protected by the unbroken Z 2 symmetry. This is also evident from the wave function. Owing to this nontrivial topological features, the wave function describes a nontrivial SPT phase. As there are three different ways to pick two generators out of the three nontrivial elements in , we can construct three different SPT wave function in this way. Therefore, this construction allows us to access all possible nontrivial phases classified using group cohomology theory. In the following sections we will present a more detailed study of this construction. Starting from a bulk Hamiltonian, we analyse its edge state and demonstrate its relation to nontrivial group cocycles. Finally, we present the field theory description of these phases [9] . Ground state wave-function on a 3D lattice Consider a 3D cubic lattice where each cube in the bulk hosts a Z 2 variable τ (big black dot in Fig. 7 ) and the Z 2 symmetry flips |0 to |1 and |1 to |0 . Each vertex in the 3D bulk hosts a variable σ (small green dot in Fig. 7 ) and the symmetry flips to and to . To define the Hamiltonian of the system, we first fix a Z 2 configuration in the cubes and define the interaction between the vertices. Start with a magnetic field in the x direction on all the spins. 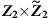Figure 7: 3D SPT model withsymmetry. Lattice model: each cube hosts aZ2variableτ(big black dot) and each vertex hosts avariableσ(small green dot) (a) a cube and the vertices around it (b) a vertex and the cubes around it. Shaded surfaces representZ2domain walls. If a vertex is on the domain wall between Z 2 configurations, modify the Hamiltonian term σ x by an extra factor of Figure 7: 3D SPT model with symmetry. Lattice model: each cube hosts a Z 2 variable τ (big black dot) and each vertex hosts a variable σ (small green dot) ( a ) a cube and the vertices around it ( b ) a vertex and the cubes around it. Shaded surfaces represent Z 2 domain walls. Full size image where n dwp is the number of domain wall pairs along the loop of all nearest neighbor spins on the same Z 2 domain wall as the original spin. If two or more Z 2 domains walls touch at the vertex, then one factor is added for each domain wall (we can pick a particular way to separate the domain walls at each vertex). Now it is easy to see that the spins form 2D nontrivial SPT states on the Z 2 domain wall. Away from the domain wall, they are polarized in the x direction. Now we include tunneling between the Z 2 configurations τ x , which in the low-energy sector of the previous Hamiltonian term not only flips the Z 2 spins but also changes the corresponding interaction pattern in its neighborhood. All these terms are local. The ground state is then unique and gapped and is the equal-weight superposition of all Z 2 configurations together with the SPT state on its domain wall and polarized spin away from its domain walls. The ground state is symmetric under the symmetry. Connecting the edge state to group cohomology Imagine that we cut the system open and expose the boundary. Note that when doing the cut, we need to be careful and not break the symmetry of the system (in particular, what we can do is double the Z 2 and spins along the cut and cut through each pair). Then on the boundary, each plaquette hosts a Z 2 variable τ i and each vertex hosts a variable σ i . It is then easy to see that on the 1D domain wall of Z 2 variables on the boundary is attached the 1D edge state of the SPT phase. The Z 2 symmetry acts by flipping the plaquettes and the symmetry acts on the σ variables living on the τ domain walls as where f ( σ i , σ i +1 ) adds a phase factor of −1 if and only if both σ i and σ i +1 are in the state . where σ z =1 for and σ z =−1 for . Here we use the symmetry convention as inref. [3] , which is equivalent to the convention used in ref. 5 . Equivalently, just like in the previous case, we can think of the 2D boundary as a system of independent degrees of freedom with one Z 2 variable τ per plaquette and one variable σ per vertex, as shown in Fig. 8 . The τ domain walls lives on the solid lines. 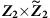Figure 8: Boundary of 3D SPT phase withsymmetry: Each plaquette hosts aZ2variableτand each vertex hosts avariableσ. Degrees of freedom within a circle are labelled by group elements of. Then, the Z 2 part of the symmetry simply acts by flipping the Z 2 variables τ i Figure 8: Boundary of 3D SPT phase with symmetry: Each plaquette hosts a Z 2 variable τ and each vertex hosts a variable σ . Degrees of freedom within a circle are labelled by group elements of . Full size image The part of the symmetry action acts by flipping the variables σ i Moreover, the symmetry also involves a phase factor of −1 whenever the τ domain wall connects two σ spins in the state. For example, at the shaded intersection shown in Fig. 8 , the phase factor is given by Such a symmetry action can be shown to be related to cocycles in a similar way as in the 2D example. In particular, in the group cohomology construction as reviewed in Supplementary Note 2 , the boundary local degrees of freedom are labelled by group elements α i of the symmetry group and the action of the symmetry operator involves two parts: first, changing the local states | α i to | αα i ; second, multiplying a phase factor given by nontrivial cocycles to each triangle of α i , α j , α k . More specifically, on the 2D boundary of 3D SPT phases, the symmetry acts as where f α ( α i , α j , α k ) is a phase factor given by the nontrivial fourth cocycle ω 4 To put the above symmetry action of into this form, we can relate each plaquette with one of its vertices (the lower right corner, for example) and think of the Z 2 and variables in this pair as labelling group element α i =( τ i , σ i ) in the symmetry group, as indicated by circles in Fig. 8 . Then, the symmetry action labelled by α = τ , σ flips the variables as Moreover, the phase factor is related to the triangle of α i =( τ i , σ i ), α j =( τ j , σ j ) and α k =( τ k , σ k ) (although it depends trivially on τ k and σ i ). Including the dependence of the phase factor on the symmetry action applied, we have Now we can reorganize the variables and check that is indeed a nontrivial four cocycle using the condition given in Supplementary Note 1 . Therefore, as discussed in Supplementary Note 2 , the state constructed in this way corresponds to a nontrivial SPT phase with symmetry and the physical features include gapless states on Z 2 domain walls on the boundary. Effective field theory description We access this 3+1D topological phase by directly constructing the 2+1 dimensional boundary. The surface is a conventional 2+1D bosonic system except in the way symmetries are implemented, which prohibit a fully symmetric, gapped and non-fractionalized surface. We expand the physical symmetry Z 2 × Z 2 to ( Z 2 × Z 2 ) × U (1). Eventually we will break the U (1) to Z 2 and identify it with one of the Z 2 generators. We begin with a bosonic field on the surface: that is charged only under the U (1) symmetry. A possible SPT surface state is to spontaneously break this U (1) symmetry by condensing this boson. Restoring the symmetry requires condensing vortices ψ of this bosonic field. However, for this to be the surface of a topological phase, the vortex transformation law must forbid a vortex condensate that preserves the remaining Z 2 × Z 2 symmetry. This can be achieved if the transformation law is projective, which implies at least a twofold degeneracy of the vortex fields hence ψ =( ψ + , ψ − ). Intuitively, one may consider the elements of the group Z 2 × Z 2 ={1, g X , g Y , g Z } as representing 180° rotations about the x , y , z axes. The projective representation is then just the spin 1/2 doublet, with the nontrivial generators represented by the Pauli matrices g a = iσ a , thus . Physical operators, which can be directly measured, do not realize symmetry in a projective fashion; however, the vortex is a non-local object and can hence transform projectively. Thus, the effective Lagrangian for the vortices is: where, by the usual duality [41] , [42] , the vortex fields are coupled to a vector potential a whose flux is the number density of b 1 bosons. Now, a vortex condensate will necessarily break symmetry since the gauge invariant combination N a = ψ † σ a ψ will acquire an expectation value. However, this transforms like a vector under rotations and will necessarily break the Z 2 × Z 2 symmetry. Thus, the theory passes the basic test for the surface state of a topological phase. This continues to be true when we break down the U(1) symmetry to Z 2 and identify it with one of the existing Z 2 symmetries. That is, the boson b 1 now transforms under the g a . This gives us three choices, which can be labelled by a = X , Y , Z , which identifies the generator that leaves b 1 invariant. Thus, the phase labelled X has b 1 →− b 1 under the generators g Y , g Z but is left invariant under g X . Even under this reduced symmetry the surface states cannot acquire a trivial gap since the condensate of b 1 continues to break some of the symmetries. Now, there are three distinct nontrivial phases implied by this construction labelled a = X , Y , Z , which, combined with the trivial phase, confirms the Z 2 × Z 2 classification of topological phases with this symmetry [1] . With this reduced symmetry, additional terms can be added to the surface Lagrangian including Δ X =−( ψ † σ x ψ cos ϕ 1 ) We would like to now verify that domain walls at the surface carry protected modes along their length. Now, consider breaking the symmetry at the surface down to a single Z 2 . When the remaining Z 2 generator is different from the one used to label the phase, we will see a protected mode is present along the surface domain walls. For example, in the set-up here where the phase is labelled by X , consider breaking the symmetry down to just the Z 2 generated by g Z . This is realized by condensing just ψ + or ψ − vortices. Consider a domain wall in the x – y plane along x =0, where for x >0 ( x <0) we have ψ + ( ψ − ) condensed. The domain wall is the region of overlap of these condensates where we have , which represents a vortex tunneling operator across the domain wall. The phase ϕ 2 is therefore conjugate to the boson phase ϕ 1 as in a Luttinger liquid. Note however the transformation law under the remaining Z 2 symmetry is: , which is the transformation law of the protected edge of the 2D Z 2 SPT phase [5] , [6] . A similar conclusion can be drawn for surface domain walls, when the remaining Z 2 symmetry is g Y . On the other hand, in this X phase, preserving the g X symmetry does not lead to protected modes since ϕ 1 is invariant under this generator and can be locked at a particular value without breaking the symmetry. Now, let us write down a 3+1D topological field theory that describes this phase. We will restrict to an abelian theory, which is not ideal given that the symmetry acts like spin rotation along orthogonal directions. Nevertheless the abelian theory gives us valuable insights. Consider the two species of bosons introduced earlier. In the phase labelled X above, the number density n 1 conjugate to ϕ 1 is invariant under all transformations, while the number density n 2 changes sign under two of them. We can always pick these to be group elements g X , g Y as above. Then we write down the following ‘BF+FF’ theory [9] : where ∈ is short for ∈ μvλσ and the indices are suppressed. Here, 2π n 1 = ∈ 0 ijk ∂ i B 1 jk is the number density of boson b 1 , and F 1 ij =∂ i a 1 j −∂ j a 1 i represents the vortex lines of boson b 1 . Thus the vector potentials a 1 are invariant under the transformations, but a 2 changes sign under g X , g Y . Therefore, the coefficient of the second term in the equation above must be quantized Θ=0, π by the usual arguments. The latter case represents the topological phase. The unusual properties of domain walls when the symmetry is broken down from Z 2 × Z 2 → Z 2 at the surface are readily deduced from this theory. A domain wall that breaks g X , g Y occurs when Θ=π→−π on the surface leads to the surface Luttinger liquid action: which describes a domain wall located along z =0, y =0, where we have replaced a 1,2 i =∂ i ϕ 1,2 . These are just the phase fields we discussed above, and in particular, under the remaining g Z transformation they are both shifted by , which is the transformation property of the nontrivial edge of a Z 2 SPT phase in 2D. In conclusion, we have presented the construction of a 2D SPT phase with symmetry by attaching Haldane chains, a 1D SPT phase with symmetry, to the Z 2 domain walls in the 2D bulk and also a 3D SPT phase with symmetry by attaching the 2D SPT state with symmetry to the domain wall of the Z 2 variables in the 3D bulk. Such a construction leads directly to the special topological feature of Z 2 domain walls on the boundary of the system: the Z 2 domain walls on the boundary carry gapless edge states of the other symmetry ( and ). We established the nontrivial SPT order in the system by relating the symmetry action on the boundary of the system to nontrivial cocycles and also demonstrated how the SPT order can be properly described using field theories. This domain wall construction also applies to 3D SPT phases with , and symmetry, including the time-reversal symmetric topological ‘superconductor’ phase, which features chiral E 8 edge modes along surface domain walls that break time-reversal symmetry. This state lies beyond the group cohomology classification. The domain wall construction of attaching d −1 dimensional SPT states of G 2 symmetry to d −1 dimensional defects in G 1 configurations was shown to be related to one term in the Künneth formula for the group cohomology of groups of the form G 1 × G 2 . Other terms in the formula may be related to attaching lower-dimensional SPT states with G 2 symmetry to lower-dimensional defects in G 1 configurations, exploring which is left to future work. A 1D SPT phase with Z 2 × Z 2 symmetry, when approached in this manner, readily suggests a parent Hamiltonian. It would be interesting to find physically well-motivated Hamiltonians that realize the higher-dimensional topological phases as well. The physical viewpoint on SPT phases described in this work may help guide such a search. Symmetry on the edge of 2D SPT with symmetry For the 2D SPT phase with symmetry, we studied one particular realization of the edge dynamics. The Hamiltonian governing the edge dynamics is given by and the Z 2 symmetry acts on the edge as while the symmetry acts as In this section, we show how to extract the low-energy effective action of the symmetry on the edge state from exact diagonalization. The Hamiltonian is an XY model (written in xz plane here) on a spin 1/2 chain and the low-energy effective theory is known to be described by the compactified free boson theory with Lagrangian The low-energy states are labelled by quantum numbers and , k =0, 1, 2…, where n 0 and label the total angular momentum and the winding number of the boson field respectively and n k and , k >0, label the left/right moving boson modes. If we normalize the ground state energy to be 0 and the first excited-state energy to be 1/4, then the energy of each low-energy state is given by and the lattice momentum p (−π/ a < p ≤π/ a ) of each state is given by where L is the total system size. n 0 is given by the conserved U (1) quantum number The boson field can be thought of as describing the direction the spin 1/2 is pointing to in the xz plane. Therefore, it corresponds to the spin state . From this, it is easy to see that the Z 2 symmetry maps ϕ to − ϕ . However, it is not easy to see the action of the time-reversal symmetry on the low-energy state because of its complicated form. In order to obtain this information, we perform exact diagonalization of the Hamiltonian, identify the n k , quantum numbers of the eigenstates from quantities like E , p , S y and find out how time-reversal symmetry acts on these states. Energy levels in the spectrum can be degenerate and p and S y allow us to partially split the degeneracy. However, states with and have the same E , p and S y . In order to tell them apart, we need to use our knowledge of the action of the Z 2 symmetry. Using the decomposition of the ϕ field where π 0 measures total angular momentum (with quantum number n 0 ), measures winding number (with quantum number ) and b k , are the annihilation operators for left/right moving boson modes (with occupation number labelled by n k and ). As the Z 2 symmetry maps ϕ to − ϕ , it maps π 0 , , , all to minus themselves. Therefore, under Z 2 symmetry action, goes to . Therefore, using the action of the Z 2 symmetry, we can further distinguish states with and fix the relative phase between them. If we want to fix the global phase factor of these two states, we can calculate the action of complex conjugation on them, which is expected to act as to . Now we are ready to look at each degenerate sector labelled by E , p , S y and see how symmetry acts on them. We discuss the first few sectors as an illustration of method. The spectrum is obtained by diagonalizing a system with 16 spin ½’s. First, the ground state with E =0, p =0, S y =0 is nondegenerate. If the phase factor is fixed such that the state is unchanged under complex conjugation, then it is invariant under both Z 2 and time-reversal symmetry. The first excited states with E =1/4 and p =0 are twofold degenerate, one with S y =1 and one with S y =−1. The two states are and . If we fix gauge such that complex conjugation acts as in this subspace and Z 2 symmetry acts as in this subspace, then time reversal acts as The third energy level at P =0 is also twofold degenerate with states and . If we fix gauge such that complex conjugation acts as in this subspace and Z 2 symmetry acts as in this subspace, then time reversal acts as The third energy level also has twofold degeneracy at P =1 with states and . If we fix gauge such that complex conjugation acts as in this subspace and Z 2 symmetry acts as in this subspace, then time reversal acts as The third energy level also has twofold degeneracy at with states and . If we fix gauge such that complex conjugation acts as in this subspace and Z 2 symmetry acts as in this subspace, then time reversal acts as . Therefore, up to finite size inaccuracy, the action of time reversal on the low energy state is consistent with to . Gauging the Z 2 symmetry In ref. 5 , Levin and Gu discussed the topological phase in d =2 protected by just Z 2 symmetry. In that case, since there is no additional symmetry, we cannot interpret the domain walls with SPT phases in d =1. However, there is a different mechanism whereby an SPT phase is generated. The domain wall ends, which are now particles, carry fractional statistics (semionic statistics in this case). In fact this is readily seen from the symmetry transformation law for the edge state of this phase ϕ 1,2 → ϕ 1,2 +π. Now, to generate a domain wall, both fields must be rotated, which is achieved by the domain wall operator . It is readily seen that D ( x ) D ( x ′)= i Sign( x − x ′) D ( x ′) D ( x ), which is the hallmark of semionic statistics in 1D. One can now gauge the Z 2 symmetry to obtain a topologically ordered state that is distinct from the regular Z 2 gauge theory [38] , [39] , [43] , [44] , [45] . In fact, the particle excitations in this theory are semions and anti-semions, and this is termed the double-semion theory. Indeed, the act of gauging the Z 2 symmetry simply implies the possibility of domain walls ending within the 2D sample. The location of these ends are just the gauge charges and fluxes. Given our experience with domain walls ending at the edge of the sample, where they have been shown to be simians, these end points are then expected to be semions. We now apply this intuition to the cased discussed here. First, consider the d =2 SPT phase with symmetry. If the Z 2 part of the symmetry is gauged, domain walls could end within the sample. We now expect these ends, which are Z 2 fluxes, to carry a spin 1/2 degrees of freedom, as shown in Fig. 9 . The gauged version of this model is similar to the one discussed in ref. 46 . From the cohomology classification we know that 2D phases with symmetry form a Z 2 × Z 2 group. Therefore, with this construction together with the nontrivial SPT phase that appears with just the Z 2 symmetry, we are able to account for all SPT phases possible in this system. 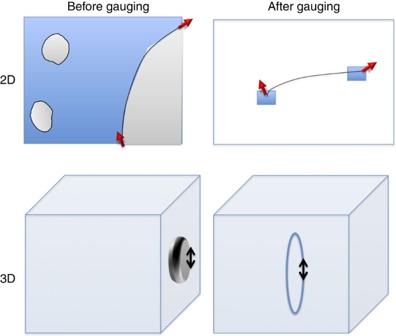Figure 9: Result of gauging theZ2symmetry: The gauge flux now allows the domain walls to terminate on them. They are point particles carrying a Kramers doublet in thed=2 system, and flux lines that carry a 1D edge state protected by the remainingglobal symmetry in thed=3 system. Figure 9: Result of gauging the Z 2 symmetry: The gauge flux now allows the domain walls to terminate on them. They are point particles carrying a Kramers doublet in the d =2 system, and flux lines that carry a 1D edge state protected by the remaining global symmetry in the d =3 system. Full size image Now consider the d =3 SPT phase with symmetry. Consider gauging g 1 the first Z 2 symmetry, but leaving the remaining engaged so it continues to act as a global symmetry. Now consider and inserting a gauge flux along a curve. It is readily seen that this flux curve will have an SPT edge state along it, specifically, the edge state of the d =2 SPT phase protected by symmetry, as shown in Fig. 9 . It can therefore be distinguished from a trivial phase, where gauging one of the Z 2 degrees of freedom does not lead to protected excitations along Z 2 flux lines. To see this, note that gauging the symmetry just means that the domain walls of g 1 ends along the flux line. However, this domain wall is now in a SPT phase. This follows from the wave function in equation (22), since the loops on the surface bounded by this curve, formed by domains of g 1 , are weighed to give a 2D Levin–Gu wave function [5] . An interesting question is the result of gauging entirely the symmetry. If we begin in the SPT phase this should lead to a Z 2 × Z 2 topological order that is distinct from the conventional one, which is described by the deconfined phase of a Z 2 × Z 2 gauge theory. Characterizing these subtle differences in topological order is left to future work. 1D SPT phase with Z 2 × Z 2 symmetry We discuss how the well-known Haldane phase in 1D can be understood within the framework of decorated domain walls. An advantage of this picture is that it leads directly to a model Hamiltonian that realizes this phase, and provides a simple rationale for the string-order parameter of this state. Consider breaking down the full SO (3) spin rotation symmetry to just Z 2 × Z 2 symmetry, which is sufficient to define this topological phase. The two Z 2 s can be modeled by a pair of Ising models σ , τ , and the ordered phases are given by or or . Consider beginning in the partially ordered phase but . Now, the domain walls of σ and the Z 2 quanta of τ are both gapped. If we condense the former, we enter the completely disordered phase. Condensing the latter leads to the completely ordered phase. However, one can consider the following scenario. What happens when we condense the bound state of σ domain wall and the τ Z 2 quanta (see Fig. 3 )? It is readily seen that this describes the SPT phase. First, since we condense domain walls of σ , the Z 2 symmetry is restored. Note, although τ quanta are condensed, they are condensed along with the domain walls, so this is not a local operator, which implies that Z 2 is also unbroken. So we have the full Z 2 × Z 2 symmetry. The easiest way to see this is the SPT phase is to consider the ‘order' parameter for this phase, which is just the condensate , where is the disorder parameter that creates/destroys a domain wall in the σ fields. So we expect long range order in: However, this is just the string order parameter for the Z 2 × Z 2 SPT phase [47] . The following space–time picture motivates why it has edge states. Consider the path integral representation in imaginary time, with a spatial boundary. Then space–time is a cylinder, the periodic direction being time. The condensate of Z 2 ‘charged’ domain walls leads to world lines that sometimes intersect the boundary. When they do, since they carry Z 2 quantum number, they flip the spin at the edge—so there must be gapless edge degrees of freedom that fluctuate in time. This picture also motivates the following Hamiltonian. First, consider a pair of decoupled Ising Models, σ and τ as shown in Fig. 3 . To enforce the binding of charge to domain walls we add the following Hamiltonian: The Hamiltonian (refs 48 , 49 ) is just a set of commuting projectors, and has a unique ground state on a system with periodic boundary conditions. However, gapless edge states appear when the system is terminated at a boundary. 3D time-reversal symmetric SPT phases The decorating domain wall picture allows us to construct nontrivial SPT phases with time-reversal symmetry also. In this section we are going to discuss 3D phases with symmetry only, symmetry and symmetry. In particular, the phase we construct with symmetry only is beyond the cohomology classification. Consider a 3D lattice with a spin 1/2 sitting in each cube. Time-reversal symmetry maps between spin up to spin down states together with the complex conjugation operation in this basis. Now we can decorate the domain wall in this spin configuration with some 2D states. First, we need to specify the orientation of the domain walls as pointing from to . Then we can put chiral states on the domain wall whose chirality matches the orientation of the domain walls. In particular, we put the Kitaev's E 8 state [50] on the domain wall, which is a bosonic 2D state with no fractional excitations in the bulk and a c − =8 edge state. After this decoration, we sum over all possible spin configurations, together with the E 8 decoration. This wave function is invariant under time-reversal symmetry, which can be seen as follows. Time reversal maps between and changing the orientation not the potision of the domain walls. At the same time, time reversal maps the E 8 state to − E 8 state with inverse chirality. Therefore, the chirality of the E 8 is always consistent with the orientation of the domain wall and the total wave function is time reversal invariant. Such a construction gives rise to a 3D SPT state with only time-reversal symmetry. Following similar arguments as in previous sections, we see that on the boundary of the system if we break time-reversal symmetry in opposite ways on neighboring regions, then the domain wall between these regions carry a chiral edge state with c − =8. This is half of what one can get in a pure 2D system without fractionalization. This is consistent with the field theory in ref. 9 . On the other hand, if time reversal symmetry is not broken, then the surface is gapless or has topological order. In fact, the surface topological state is that with three fermions [21] , [22] , which cannot be realized in pure 2D system with time-reversal symmetry. Similar construction applies to 3D SPT phases with and symmetry. In 2D with U (1) and SO (3) symmetry, there is an integer class of SPT phases with even-integer-quantized charge or spin Hall conductance [8] , [13] , [14] , [45] . Similar to the construction above, we can put the first nontrivial phase in this class to the domain wall of time reversal. The Hall conductance chirality should match the domain wall orientation. By summing over all spin configurations, we obtain a state with both time reversal and U (1) or SO (3) symmetry. One signature of the state would be even-integer-quantized Hall conductance on the time reversal domain wall on the 2D surface of the system. Relation to Künneth formula for group G = G 1 × G 2 If a group G is the direct product of two subgroups G = G 1 × G 2 , then the Künneth formula for the group cohomology of G can be written as [38] which says that cohomology groups of G in d +1 dimension can be obtained from cohomology groups of G 1 and G 2 in lower dimensions. Owing to the relation between cohomology groups and SPT phases, this implies that SPT phases with G symmetry in d dimension can be constructed from SPT phases with G 1 and G 2 symmetry in lower dimensions. When k =0, the term in the formula is which means that some SPT phases with symmetry G in d dimension are just SPT phases with symmetry G 2 in d dimension. When k = d +1, the term in the formula is which means that some SPT phases with symmetry G in d dimension are just SPT phases with symmetry G 1 in d dimension. Our domain wall construction correspond to the term with k =1 ( G 2 , U (1)) labels SPT phases with G 2 symmetry in d −1 dimensions. If ( G 2 , U (1))= M ( M = Z n , Z for example), then the term becomes ( G 1 , M ), which labels 1D representations of G 1 using M coefficient. Therefore, this term says that some d dimensional SPT phase with G symmetry can be obtained from d −1 dimensional SPT phases with G 2 symmetry and 1D representation of G 1 with M coefficient. Our domain wall construction provides a physical interpretation of the above statement. With discrete G 1 group, as in the cases we are interested in, consider a d dimensional configuration with group elements in G 1 . The domain walls are then also labelled by group elements given by the difference of the group elements on the two sides of the wall. Then on the d −1 dimensional domain wall labelled by g 1 , we can choose to put d −1 dimensional SPT phases from the class M . Our choice should be consistent with the fusion rules of the domain walls. That is, the phases m a and that we choose to put onto domain walls and should combine into the phase m ab , which we put onto the domain wall labelled by . In other words, this correspond to a 1D representation of group G 1 in coefficient M . Therefore, the term with k =1 in the formula 47 corresponds exactly to our domain wall construction. Note that this formula also gives the condition of when such domain wall construction can be consistent. In particular, when putting the d −1 dimensional SPTs onto the domain walls, we need to put them according to the corresponding 1D representation of G 1 in M . Suppose we have M = Z 3 , then putting the first nontrivial one onto a Z 2 domain wall is not allowed because two Z 2 domain walls can merge to trivial and so should the corresponding SPTs. Terms with higher k ’s would correspond to constructing d dimensional SPT phases with G symmetry by putting d−k dimensional SPT phases with G 2 symmetry onto d−k dimensional defects in G 1 configurations. How to cite this article: Chen, X. et al. Symmetry-protected topological phases from decorated domain walls. Nat. Commun. 5:3507 doi: 10.1038/ncomms4507 (2014).